Existence of long-lasting experience-dependent plasticity in endocrine cell networks Experience-dependent plasticity of cell and tissue function is critical for survival by allowing organisms to dynamically adjust physiological processes in response to changing or harsh environmental conditions. Despite the conferred evolutionary advantage, it remains unknown whether emergent experience-dependent properties are present in cell populations organized as networks within endocrine tissues involved in regulating body-wide homeostasis. Here we show, using lactation to repeatedly activate a specific endocrine cell network in situ in the mammalian pituitary, that templates of prior demand are permanently stored through stimulus-evoked alterations to the extent and strength of cell–cell connectivity. Strikingly, following repeat stimulation, evolved population behaviour leads to improved tissue output. As such, long-lasting experience-dependent plasticity is an important feature of endocrine cell networks and underlies functional adaptation of hormone release. The possession of long-term experience-dependent plasticity by biological systems allows organisms to dynamically change their physiology to suit the prevailing environmental conditions. At the cellular level, this process is classically associated with the immune system, allowing heightened and more effective lymphocyte responses following re-encounter with antigen [1] , [2] . At the tissue level, experience-dependent changes are best characterized in the brain. Following stimulus, the connectivity of neurons is modified through permanent changes in the strength and number of synaptic contacts [3] , [4] , [5] , improving functional outcome in response to repeated challenge [6] , [7] . Given the evolutionary and physiological advantages conferred by functional adaptation, we reasoned that experience-dependent plasticity may also represent an inherent property of cells that populate tissues involved in mounting large-scale homeostatic responses. The mammalian pituitary gland represents an ideal model organ with which to test this hypothesis as it consists of endocrine cells arranged as networks [8] , [9] , [10] , [11] , a prerequisite for adaptive processes [12] , [13] , [14] , and regulates multiple physiological functions through the secretion of hormone. Therefore, to determine whether endocrine cell networks possess emergent experience-dependent properties, we decided to use lactation as a demand with which to repeatedly and selectively stimulate activity of pituitary lactotrophs. The secretion of prolactin (PRL) by these cells drives a range of responses crucial for nurture of offspring, including mammary gland development/output [15] and neurogenesis [16] , [17] , the latter being essential for the display of maternal behaviour [18] . Profound and lasting changes in lactotroph population function would therefore be expected to represent an essential element of physiological adaptation when females experience one or more lactations (herein termed parity). Here, using two-photon calcium imaging in combination with mathematical analyses to discriminate cell population interactivity, we show that endocrine cell networks in situ undergo marked functional plasticity in response to demand. Poststimulus, the cell population faithfully stores a functional template through permanent morphological and gap junction (GJ)-driven changes to the extent and strength of network connectivity. Subsequently, repeat challenge with the same stimulus is met with evolved network dynamics and improved tissue output. As such, these findings show that long-lasting experience-dependent plasticity is a key feature of endocrine cell populations organized within the mammalian pituitary gland, and permits functional adaptation of hormone secretion. Endocrine cells display functional plasticity in situ To provide an activity index of both population function [8] , [19] , [20] and calcium (Ca 2+ )-dependent hormone exocytosis [21] (the major pituitary output), we measured multi-cellular Ca 2+ signals emanating from lactotrophs in situ within pituitary slices derived from PRL-DsRed mice [22] . Population functional connectivity (FC) maps were constructed based on the location of significantly correlated cell pairs (that is, cells with related activity profiles). In nulliparas (virgins), low levels of PRL secretion (12.3±2.5 ng ml −1 ) were associated with some correlated cell–cell communication due to firing of spontaneous short-lived Ca 2+ spikes ( Fig. 1a and i ; Supplementary Movie 1 ). The connection distribution was best fitted with a power-law, indicating that a few cells host the majority of links, functionally connecting distant ensembles ( Fig. 1g; n =28 slices/18 animals) [23] , [24] . During lactation in primiparas (first lactation), the emergence of long-lasting Ca 2+ plateaus ( Fig. 1b and e ; Supplementary Movie 2 ) was accompanied by dramatic increases in basal coactivity ( Fig. 1b ), proportion of correlated cell pairs ( Fig. 1f ) and circulating PRL concentrations (102.5±21.7 ng ml −1 ; P <0.05 versus nulliparas; Fig. 1i ). The extra correlated cell pairs were re-distributed as new nodes, each with a similar number of connections ( Fig. 1b and g ), as evidenced by a reduction in the mean power-law exponent value ( γ ), a quantitative descriptor of the characteristic connection distribution ( γ =1.57±0.39 versus 1.09±0.05, nullipara versus primipara, respectively; n =16 slices/10 animals, P <0.01; Fig. 1h ). Highly connected cells (>40% links) were characterized by low frequency, regular Ca 2+ plateaus and their location was dynamic due to spontaneous transitions between Ca 2+ -spiking states ( Supplementary Fig. S1a and b ). As correlated cell behaviour and FC were maintained over the long term ( Supplementary Fig. S1c and d ), this finely tuned readjustment of Ca 2+ -spike patterning may provide an important means to maintain population communication in the face of node failure (for example, fatigue/apoptosis). 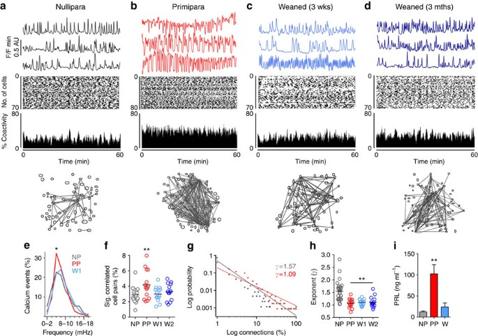Figure 1: Lactation induces alterations in lactotroph population functional connectivity. (a) Nullipara (NP): top panel shows representative cytosolic Ca2+traces in NP lactotrophs (AU, arbitrary units). Cells are spontaneously active and fire short-lived Ca2+spikes. Middle panels show binarized Ca2+traces for all cells represented as a raster plot and % coactivity plotted as a function of time. Note the low levels of cell-cell coactivity. Bottom panel shows a functional connectivity (FC) map depicting the location of significantly (Sig.) correlated cell pairs. (b) Panels as forabut for primiparas (PP). Ca2+-spiking activity increases with demand and displays long-lasting plateaus. Raster plot shows regular Ca2+spiking, which is highly coordinated at the cell-pair level. Cell–cell coactivity is increased. FC map showing densification. (c) Panels as forabut for 3-week weaned dams (W1). Ca2+-spiking activity returns to nullipara levels. Raster plot and coactivity are identical to that observed in nulliparas. A lactating-like FC is retained. (d) All panels as incbut for 3-month weaned dams (W2). (e) Mean Ca2+-spiking frequency is lower in primiparas versus nulliparas due to a longer time spent 'on'. Postweaning, frequency returns to nullipara levels (*P<0.05, PP versus NP; two-way analysis of variance;n=13–18 slices from at least four animals) (f) There is a transient increase in % correlated cell pairs during lactation (**P<0.01 versus NP; Kruskal–Wallis test). Values represent mean±s.e.m. (n=14–17 slices from at least five animals). (g) Probability plot showing proportion of connections hosted by cells from the imaged population of nulliparas (grey) and primiparas (red). Solid lines represent power-laws constructed using the mean exponent (γ)-value and superimposed over the pooled data set (n=28 slices). (h) The mean power-law exponent (γ)-value is lower in primiparas versus nulliparas as correlated cell pairs are laid down in the form of new nodes, each with a similar connection number.γ-Value remains low postweaning due to the retention of a lactating-like FC (**P<0.01 versus NP; Kruskal–Wallis test;n=14–28 slices from at least five animals). (i) Prolactin (PRL) concentrations increase during lactation (**P<0.01 versus NP; Kruskal–Wallis test;n=11–19 animals). Values represent mean±s.e.m. Mths, months; Wks, weeks. Figure 1: Lactation induces alterations in lactotroph population functional connectivity. ( a ) Nullipara (NP): top panel shows representative cytosolic Ca 2+ traces in NP lactotrophs (AU, arbitrary units). Cells are spontaneously active and fire short-lived Ca 2+ spikes. Middle panels show binarized Ca 2+ traces for all cells represented as a raster plot and % coactivity plotted as a function of time. Note the low levels of cell-cell coactivity. Bottom panel shows a functional connectivity (FC) map depicting the location of significantly (Sig.) correlated cell pairs. ( b ) Panels as for a but for primiparas (PP). Ca 2+ -spiking activity increases with demand and displays long-lasting plateaus. Raster plot shows regular Ca 2+ spiking, which is highly coordinated at the cell-pair level. Cell–cell coactivity is increased. FC map showing densification. ( c ) Panels as for a but for 3-week weaned dams (W1). Ca 2+ -spiking activity returns to nullipara levels. Raster plot and coactivity are identical to that observed in nulliparas. A lactating-like FC is retained. ( d ) All panels as in c but for 3-month weaned dams (W2). ( e ) Mean Ca 2+ -spiking frequency is lower in primiparas versus nulliparas due to a longer time spent 'on'. Postweaning, frequency returns to nullipara levels (* P <0.05, PP versus NP; two-way analysis of variance; n =13–18 slices from at least four animals) ( f ) There is a transient increase in % correlated cell pairs during lactation (** P <0.01 versus NP; Kruskal–Wallis test). Values represent mean±s.e.m. ( n =14–17 slices from at least five animals). ( g ) Probability plot showing proportion of connections hosted by cells from the imaged population of nulliparas (grey) and primiparas (red). Solid lines represent power-laws constructed using the mean exponent ( γ )-value and superimposed over the pooled data set ( n =28 slices). ( h ) The mean power-law exponent ( γ )-value is lower in primiparas versus nulliparas as correlated cell pairs are laid down in the form of new nodes, each with a similar connection number. γ -Value remains low postweaning due to the retention of a lactating-like FC (** P <0.01 versus NP; Kruskal–Wallis test; n =14–28 slices from at least five animals). ( i ) Prolactin (PRL) concentrations increase during lactation (** P <0.01 versus NP; Kruskal–Wallis test; n =11–19 animals). Values represent mean±s.e.m. Mths, months; Wks, weeks. Full size image Templates of prior demand persist at the population level To test whether FC was plastic, lactotroph population activity was measured following cessation of demand. Three weeks following weaning, a lactating-like FC was still present ( γ =1.10±0.03; P <0.01 versus nullipara; n =14 slices/5 animals, Fig. 1c and h ) despite return of Ca 2+ -spiking activity ( Fig. 1c and e ), correlated cell pair number ( Fig. 1f ) and PRL concentrations to nullipara levels ( Fig. 1i ). This was not due to advancing age or acute remodelling events as correlated cell pairs were distributed identically in nulliparas of similar age to weaned animals ( Supplementary Fig. S2a ), and a lactating-like FC remained even 3 months postweaning (γ=1.09±0.05; P <0.01 versus nulliparas; n =16 slices/5 animals, Fig. 1d and h ). To elucidate whether the characteristic FC's observed in primiparas and weaned dams were due to suckling stimulus, or simply imprinted on the system during pregnancy, experiments were performed using animals exposed to reduced lactational demand by altering the number of suckling pups immediately postpartum. By leaving only three pups from an original of eight ( Supplementary Fig. S2b ), FC was identical to that seen in nulliparas ( γ =1.55±0.07 versus 1.41±0.09, nulliparas versus primiparas reduced, respectively; nonsignificant, NS; n =12 slices/4 animals) and remained similar following weaning ( γ =1.37±0.03; n =11 slices/3 animals, Fig. 2a and b ). Therefore, suckling promotes the changes in FC that are observed during lactation and retained in weaned dams. 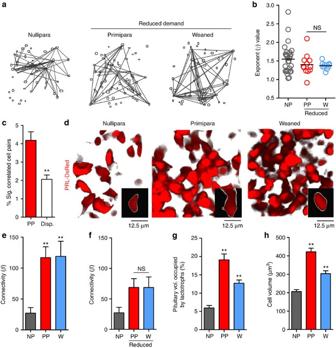Figure 2: Suckling promotes lactotroph population functional connectivity through changes in structural connectivity. (a) Functional connectivity does not change in primiparas or weaned dams subjected to lactation with reduced suckling stimulus. (b) Confirming (a) statistically, power-law exponent (γ)-value for primiparas (PP) and weaned (W) dams subjected to reduced demand is similar to that observed in nulliparas (NP; NS, nonsignificant versus NP; Kruskal–Wallis test,n=11–12 from at least three animals). (c) Correlated cell–cell behaviour is impaired in primiparas when tissue structure is disrupted (Disp.; **P<0.01; Mann–WhitneyU-test,n=12 from four animals). Values represent mean±s.e.m. (d) Lactotrophs are organized into a three-dimensional network. Structural connectivity is low in nulliparas (left panel), but increases in primiparas (middle panel). Following weaning, connectivity is maintained despite cessation of stimulus (right panel). Insets are typical cell profiles. (e) To directly correlate structural (SC) and functional (FC) connectivity, three-dimensional reconstructions were acquired of the lactotroph network subjected to Ca2+imaging. Postanalysis of connectivity (β) reveals an increase in SC in primiparas that reflects heightened FC. Postweaning, high levels of SC persist (**P<0.01 versus NP; Kruskal–Wallis test,n=12–14 slices from at least five animals). Values represent mean±s.e.m. (f) As fore, but for primiparas and weaned dams subjected to reduced demand. Note that SC was no different to nulliparas (NS, nonsignificant versus NP; Kruskal–Wallis test,n=9–11 slices from three animals). Values represent mean±s.e.m. (g) Pituitary volume occupied by lactotrophs increases in primiparas versus nulliparas and this persists following weaning (**P<0.01 versus NP; Kruskal–Wallis test,n=15–21 image stacks from three animals). Values represent mean±s.e.m. (h) Lactotroph network density and plasticity are driven by anin situincrease in cell volume as calculated by single-cell rendering of image stacks (**P<0.01 versus NP; Kruskal–Wallis test,n=62 cells from three animals). Values represent mean±s.e.m. Sig. significant. Figure 2: Suckling promotes lactotroph population functional connectivity through changes in structural connectivity. ( a ) Functional connectivity does not change in primiparas or weaned dams subjected to lactation with reduced suckling stimulus. ( b ) Confirming ( a ) statistically, power-law exponent ( γ )-value for primiparas (PP) and weaned (W) dams subjected to reduced demand is similar to that observed in nulliparas (NP; NS, nonsignificant versus NP; Kruskal–Wallis test, n =11–12 from at least three animals). ( c ) Correlated cell–cell behaviour is impaired in primiparas when tissue structure is disrupted (Disp. ; ** P <0.01; Mann–Whitney U -test, n =12 from four animals). Values represent mean±s.e.m. ( d ) Lactotrophs are organized into a three-dimensional network. Structural connectivity is low in nulliparas (left panel), but increases in primiparas (middle panel). Following weaning, connectivity is maintained despite cessation of stimulus (right panel). Insets are typical cell profiles. ( e ) To directly correlate structural (SC) and functional (FC) connectivity, three-dimensional reconstructions were acquired of the lactotroph network subjected to Ca 2+ imaging. Postanalysis of connectivity ( β ) reveals an increase in SC in primiparas that reflects heightened FC. Postweaning, high levels of SC persist (** P <0.01 versus NP; Kruskal–Wallis test, n =12–14 slices from at least five animals). Values represent mean±s.e.m. ( f ) As for e , but for primiparas and weaned dams subjected to reduced demand. Note that SC was no different to nulliparas (NS, nonsignificant versus NP; Kruskal–Wallis test, n =9–11 slices from three animals). Values represent mean±s.e.m. ( g ) Pituitary volume occupied by lactotrophs increases in primiparas versus nulliparas and this persists following weaning (** P <0.01 versus NP; Kruskal–Wallis test, n =15–21 image stacks from three animals). Values represent mean±s.e.m. ( h ) Lactotroph network density and plasticity are driven by an in situ increase in cell volume as calculated by single-cell rendering of image stacks (** P <0.01 versus NP; Kruskal–Wallis test, n =62 cells from three animals). Values represent mean±s.e.m. Sig. significant. Full size image To investigate whether these alterations were due to the well-characterized changes in dopamine tone that occur during lactation and allow heightened lactotroph activity in response to suckling [25] , [26] , nulliparas were treated for 10 days with the dopamine-2-receptor antagonist, metoclopramide. Following treatment, no differences in FC ( Supplementary Fig. S3a and b ) were observed versus nulliparas ( n =12 slices/5 animals). By contrast, the same treatment caused large increases in Ca 2+ -spiking frequency ( Supplementary Fig. S3c ) and PRL concentrations ( Supplementary Fig. S3d ). Therefore, D2-antagonism increases lactotroph output in a network-independent manner through effects on single-cell Ca 2+ -spiking activity, and dopamine-alone is unlikely to account for suckling-induced changes in FC. Nonetheless, postweaning, the return of high levels of dopamine presumably balances enhanced cell-network connectivity by suppressing lactotroph Ca 2+ -spiking activity to maintain low PRL output [27] . Structural plasticity facilitates storage of wiring patterns Next, we assessed whether the changes in FC induced by maternal experience were driven by permanent alterations in structural connectivity (SC). Tissue organization of cells was critical for coherent communication during lactation as enzymatic dissociation of glands substantially decreased correlated cell behaviour ( n =12 recordings/4 animals; Fig. 2c ), despite retention of plateauing Ca 2+ activity ( Supplementary Fig. S4 ). Imaging of fixed tissue revealed the existence of a topologically organized lactotroph-network pervading the gland that, at higher magnifications, appeared to be more highly connected in primiparas and weaned dams ( Fig. 2d ). To directly correlate FC with SC, online three-dimensional reconstructions of the lactotroph population subjected to Ca 2+ imaging were captured. Compared with nulliparas, SC was increased in primiparas and this was maintained in weaned dams ( Fig. 2e ). SC was directly influenced by suckling as it was decreased in animals exposed to reduced demand ( Fig. 2f ). As expected, this was unrelated to suckling-induced changes in dopamine tone, as SC was not altered in metoclopramide-treated animals ( β =35.29±9.19, NS versus nullipara; n =12 slices/5 animals). The increased connectivity during and after lactation could be accounted for by a persistent increase in the organ volume occupied by lactotrophs ( Fig. 2g ), the result of an in situ increase in cell size ( Fig. 2h ). Previous studies have indicated that, in the lactating murine pituitary gland, lactotroph hypertrophy occurs in the absence of hyperplasia [28] . Changes in structure induce improved cell–cell communication As a change in SC does not necessarily imply reciprocal alterations in the strength of information transfer through the lactotroph network, the degree of cell–cell communication was investigated. GJs were targeted as they are widely implicated in cell signalling in the pituitary [29] . Injection of a GJ-permeable dye into lactotrophs revealed that functional GJ coupling was present before, during and after demand ( Fig. 3a , top panel). However, the extent of dye coupling was greatest in primiparas and weaned dams versus nulliparas, and transfer could be reduced by 18-α-glycyrrhetinic acid (AGA), a GJ blocker ( Fig. 3a–c; n =14–39 injected cells, 3–5 animals for each condition). It is likely that the lactotroph network provides a structural conduit for the observed FC patterns as the majority of GJ contacts were homotypic between lactotrophs. This was demonstrated by both dye-coupling studies (70.5±1.4% probability of dye transfer to a lactotroph, n =94 injected cells, 13 animals; Fig. 3d ) and morphological identification of intercellular junctions on electron micrographs ( Fig. 3e and f ). Furthermore, continuous three-dimensional paths of homotypic cell–cell contacts were traced between correlated cell pairs, hinting that GJ signalling through structurally interconnected chains of lactotrophs could conceivably account for the observed FC patterns ( Supplementary Fig. S5a ). Reinforcing this was the observation that dye-coupled lactotrophs were often located in different focal planes (see Methods ). Other pituitary cell networks may also be implicated in functionally linking lactotrophs over long distances, especially in the nullipara lactotroph network where GJ coupling was lower and proportionally more heterotypic contacts with growth hormone (GH) and folliculostellate (FS) cells were present ( Fig. 3e ; Supplementary Fig. S5b and c ). The latter cell type has previously been shown to electrically propagate signals over a 1-mm range [30] . 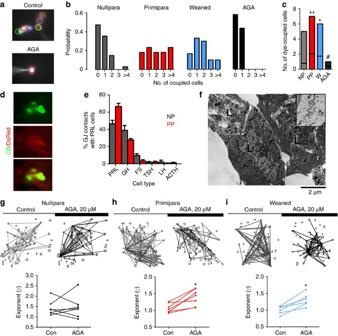Figure 3: Homotypic lactotroph–lactotroph GJ contacts underlie observed functional connectivity patterns. (a) Injection of a gap junction (GJ)-permeable dye into lactotrophs of lactating animals reveals GJ coupling (top panel; Control) that is blocked by pre-exposure to 18-α-glycerrhitinic acid (AGA) 20 μM (bottom panel; AGA). Images were acquired with an epifluorescence microscope, and passage of dye to lactotrophs in different focal planes was frequently observed. (b) Lactotrophs are GJ coupled under all states tested, but there is increased probability of GJ transfer in primiparas (red bars,n=39) and weaned dams (blue bars,n=30) versus nulliparas (grey bars,n=25). AGA application (black bars,n=14) reduces the probability of GJ transfer between lactotrophs of primiparas. As fora, images were acquired with an epifluorescence microscope. (c) Floating bar plot (displaying min–max and median values) showing significant increases in GJ coupling in primiparas (PP) and weaned animals (W) that are abolished by AGA (*P<0.05 and **P<0.01 versus NP;##P<0.01 versus PP; Kruskal–Wallis test,nas forb). (d) Following injection of Cascade Blue (CB) (pseudocoloured in green, top panel) into lactotrophs (DsRed, middle panel), GJ transfer is homotypic (bottom panel). (e) Electron microscopic identification of intercellular junctions between lactotrophs (PRL) and other pituitary cell types. The majority of contacts are homotypic between lactotrophs in both nulliparas and primiparas, but proportionally more contacts with folliculostellate (FS) cells are observed in the former (n=40 observations). Values represent mean±s.e.m. (f) Representative electron micrograph of homotypic contacts between lactotrophs (L). Inset is a higher magnification (×2.5; scale bar, 800 nm) view of a junction connecting two lactotrophs. (g) Application of AGA does not affect functional connectivity (FC) in nulliparas (top panels). Power-law exponent (γ) value, and thus FC, is unchanged following application of AGA to nullipara slices (connected points represent before and during treatment for each trial,n=7 slices; bottom panel). (h) Application of AGA alters FC in primiparas (top panels). For all trials,γ-value increases following application of AGA to primipara slices indicating re-emergence of a nullipara-like FC (*P<0.05 versus control (Con); Wilcoxon signed-rank test,n=7 slices; bottom panel). (i) As forgbut for weaned dams (*P<0.05 versus control (Con); Wilcoxon signed‐rank test,n=6 slices). Figure 3: Homotypic lactotroph–lactotroph GJ contacts underlie observed functional connectivity patterns. ( a ) Injection of a gap junction (GJ)-permeable dye into lactotrophs of lactating animals reveals GJ coupling (top panel; Control) that is blocked by pre-exposure to 18-α-glycerrhitinic acid (AGA) 20 μM (bottom panel; AGA). Images were acquired with an epifluorescence microscope, and passage of dye to lactotrophs in different focal planes was frequently observed. ( b ) Lactotrophs are GJ coupled under all states tested, but there is increased probability of GJ transfer in primiparas (red bars, n =39) and weaned dams (blue bars, n =30) versus nulliparas (grey bars, n =25). AGA application (black bars, n =14) reduces the probability of GJ transfer between lactotrophs of primiparas. As for a , images were acquired with an epifluorescence microscope. ( c ) Floating bar plot (displaying min–max and median values) showing significant increases in GJ coupling in primiparas (PP) and weaned animals (W) that are abolished by AGA (* P <0.05 and ** P <0.01 versus NP; ## P <0.01 versus PP; Kruskal–Wallis test, n as for b ). ( d ) Following injection of Cascade Blue (CB) (pseudocoloured in green, top panel) into lactotrophs (DsRed, middle panel), GJ transfer is homotypic (bottom panel). ( e ) Electron microscopic identification of intercellular junctions between lactotrophs (PRL) and other pituitary cell types. The majority of contacts are homotypic between lactotrophs in both nulliparas and primiparas, but proportionally more contacts with folliculostellate (FS) cells are observed in the former ( n =40 observations). Values represent mean±s.e.m. ( f ) Representative electron micrograph of homotypic contacts between lactotrophs (L). Inset is a higher magnification (×2.5; scale bar, 800 nm) view of a junction connecting two lactotrophs. ( g ) Application of AGA does not affect functional connectivity (FC) in nulliparas (top panels). Power-law exponent ( γ ) value, and thus FC, is unchanged following application of AGA to nullipara slices (connected points represent before and during treatment for each trial, n =7 slices; bottom panel). ( h ) Application of AGA alters FC in primiparas (top panels). For all trials, γ -value increases following application of AGA to primipara slices indicating re-emergence of a nullipara-like FC (* P <0.05 versus control (Con); Wilcoxon signed-rank test, n =7 slices; bottom panel). ( i ) As for g but for weaned dams (* P <0.05 versus control (Con); Wilcoxon signed‐rank test, n =6 slices). Full size image Whereas exogenous application of AGA did not alter FC when applied to slices from nulliparas ( Fig. 3g ), it resulted in re-emergence of a nullipara-like FC when applied to slices from primipara ( Fig. 3h ) and weaned dams ( Fig. 3i ), supporting involvement of GJ's in promoting FC. Consistent with a role of homotypic GJ contacts in facilitating the increased number of long-range connections detected in primiparas was the observation that AGA significantly reduced the average distance between correlated cell pairs ( Supplementary Fig. S6 ). The role of alternative signalling –modalities, such as diffusible factors, were excluded on the basis that their diffusion patterns are not consistent with the observed FC's [31] . Long-distance entrainment of lactotroph network activity As voltage-gated Ca 2+ currents participate in action potential generation in endocrine cells [32] , network-wide Ca 2+ signals were recorded while simultaneously subjecting individual cells to depolarizing voltage pulses to assess whether lactotrophs were capable of electrically entraining their activity. Using this technique, we were able to detect long-distance propagation of Ca 2+ signals (median lag=1.06±1.72 s), which encompassed multiple lactotrophs following cell stimulation (28 trials/5 animals; Fig. 4a ; Supplementary Movie 3 ). The number of responsive cells varied greatly, presumably reflecting the connectivity of the randomly targeted lactotroph (range=1–16 cells), and signals transferred rapidly (instantaneous conduction velocity=147.1±36 μm s −1 ) with minimal diminishment of Ca 2+ -spike amplitude as a function of distance ( R 2 =0.0296; estimated from a two-dimensional optical slice of the network). In all cases, entrainment was due to intercellular communication through GJ's, as propagation could be blocked using AGA (27 trials/4 animals; Fig. 4b ). Neighbouring cells did not always activate, providing further evidence that lactotrophs may be GJ coupled through chains of cells located outside the focal plane. The Euclidean distances between entrained cells reflected that calculated on the basis of correlated Ca 2+ -spiking activity (range=9.2–205.0 μm), strengthening the notion that lactotrophs can communicate in three-dimensions over long distances via GJ's to coordinate activity and form functional links. 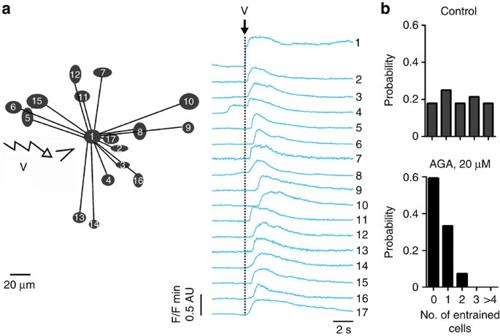Figure 4: Entrainment of lactotroph activity involves GJ-mediated intercellular communication. (a) Following application of a 500 ms depolarizing voltage (V) pulse (onset marked with a black dashed line) onto individual DsRed-positive cells within slices from weaned animals, lactotrophs located at distance (left panel) respond with rises in intracellular Ca2+levels (right panel). The stimulating pipette was touching cell 1 (left panel; triangle) and, for the sake of clarity, only cells that responded with intracellular Ca2+rises are represented on the connectivity map (AU, arbitrary units). (b) Histograms showing probability of lactotroph entrainment in the absence (top panel;n=28 recordings from five animals) and the presence (bottom panel;n=27 recordings from four animals) of 18-alpha-glycerrhitinic acid (AGA). Note that application of AGA severely impedes cell–cell signal propagation. In all cases, to allow accurate discrimination of entrainment, lactotroph network activity was dampened by constant perfusion with dopamine (100 nM). Figure 4: Entrainment of lactotroph activity involves GJ-mediated intercellular communication. ( a ) Following application of a 500 ms depolarizing voltage (V) pulse (onset marked with a black dashed line) onto individual DsRed-positive cells within slices from weaned animals, lactotrophs located at distance (left panel) respond with rises in intracellular Ca 2+ levels (right panel). The stimulating pipette was touching cell 1 (left panel; triangle) and, for the sake of clarity, only cells that responded with intracellular Ca 2+ rises are represented on the connectivity map (AU, arbitrary units). ( b ) Histograms showing probability of lactotroph entrainment in the absence (top panel; n =28 recordings from five animals) and the presence (bottom panel; n =27 recordings from four animals) of 18-alpha-glycerrhitinic acid (AGA). Note that application of AGA severely impedes cell–cell signal propagation. In all cases, to allow accurate discrimination of entrainment, lactotroph network activity was dampened by constant perfusion with dopamine (100 nM). Full size image Tissue output is improved in an experience-dependent manner Finally, we hypothesized that experience-dependent plasticity would allow improved lactotroph network behaviour in response to repeated stimulus, as has been shown at the cellular level for circulating lymphocytes [1] , [2] and at the tissue level for neurons belonging to the brain [6] , [7] . To test this, network behaviour was analysed following induction of a second lactation. In multiparas (second lactation), no further changes in pituitary volume occupied by lactotrophs (21.0±0.9%, NS versus primipara), SC (β=162.4±26.0, NS versus primipara) or cell volume (453±30.4 μm 3 , NS versus primipara) were evident. A densely wired lactotroph population was recalled through recruitment of extra correlated cell pairs (4.46±0.39 versus 2.99±0.25% significantly correlated cell pairs, multipara and weaned, respectively; P <0.01) to the FC template stored by weaned dams (γ=1.02±0.04, NS versus weaned; n =16 slices/6 animals, Fig. 5a ). By contrast to primiparas, this was associated with the GJ-driven emergence of synchronized cell activity ( Fig. 5a ), as indicated by a Gaussian distribution of intercoactivity intervals with a peak of 115 s ( Fig. 5b ), which could be abolished by application of AGA ( Fig. 5c; Supplementary Movie 4 ). Strikingly, this generated even higher levels of hormone secretion compared with the first lactation (266.2±64.1 ng ml −1 , P <0.01 versus primiparas; Fig. 5e ). To investigate if disruption of FC during the first lactation impaired the potentiated network response observed following repeat demand, primiparas exposed to reduced suckling stimulus were subjected to a second lactation. In these animals, network dynamics and PRL secretion were similar to that observed in primiparas, suggesting that changes occurring during the first lactation are obligatory for increasing functional performance during the second lactation ( n =13 slices/5 animals, Fig. 5d and e; Supplementary Movie 5 ). High PRL levels were not due to the advanced age of multiparas relative to primiparas as no relationship between PRL concentrations and age was detected during the first lactation ( Supplementary Fig. S7a ). It is unlikely that there were differences in suckling stimulus between primiparas and multiparas, as average litter size was identical in both sets of animals ( Supplementary Fig. S7b ). Therefore, despite being exposed to similar stimulus, the lactotroph population is able to display enhanced functional performance and output during the second lactation. 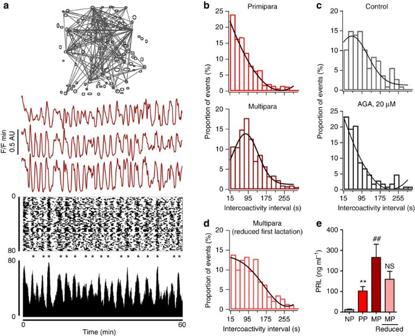Figure 5: Lactotroph network displays evolved behaviour and output following repeat stimulus. (a) Functional connectivity (FC) map shows that connection distribution is similar in multiparas and primiparas (top panel). Middle panels show representative Ca2+traces in lactotrophs of multiparas (second lactation; MP) with spontaneous Ca2+-spiking activity in lactotrophs identical to that observed in primiparas (AU, arbitrary unit), and a raster plot shows regular Ca2+ spiking that is distributed homogeneously over time at the population level. Distinct peaks of cell–cell coactivity are observed due to emergence of synchrony (*=peak of coactivity over a 95% significance threshold; bottom panel). (b) Probability histogram of intercoactivity intervals for primiparas (top panel) and multiparas (bottom panel). Note that peaks of coactivity due to cell synchrony are only observed in multiparas, as demonstrated by a Gaussian distribution of intercoactivity intervals centred on 115s (n=16–19 slices from at least six animals). (c) Probability histogram of intercoactivity intervals for multiparas exposed to Control and 18-alpha-glycerrhitinic acid (AGA) 20 μM. GJ blockade with AGA results in reversion to a primipara intercoactivity interval distribution due to abolition of cell synchrony (n=8 slices from three animals). (d) Probability histogram of intercoactivity intervals for multiparas suckled by a reduced number of pups during the first lactation. Prior exposure to a reduced suckling stimulus disrupts appearance of coactivity peaks in multiparas as shown by a non-Gaussian distribution of intercoactivity intervals (n=13 slices from five animals). (e) Tissue output in the form of prolactin (PRL) secretion markedly increases as a function of lactational experience (**P<0.01 versus nullipara (NP),##P<0.01 versus primipara (PP); Kruskal–Wallis test) and this can be reversed by exposing multiparas to reduced demand during the first lactation (NS, nonsignificant versus PP; Kruskal–Wallis test;n=6–19 animals). Values represent mean±s.e.m.± Figure 5: Lactotroph network displays evolved behaviour and output following repeat stimulus. ( a ) Functional connectivity (FC) map shows that connection distribution is similar in multiparas and primiparas (top panel). Middle panels show representative Ca 2+ traces in lactotrophs of multiparas (second lactation; MP) with spontaneous Ca2+-spiking activity in lactotrophs identical to that observed in primiparas (AU, arbitrary unit), and a raster plot shows regular Ca2+ spiking that is distributed homogeneously over time at the population level. Distinct peaks of cell–cell coactivity are observed due to emergence of synchrony (*=peak of coactivity over a 95% significance threshold; bottom panel). ( b ) Probability histogram of intercoactivity intervals for primiparas (top panel) and multiparas (bottom panel). Note that peaks of coactivity due to cell synchrony are only observed in multiparas, as demonstrated by a Gaussian distribution of intercoactivity intervals centred on 115s ( n =16–19 slices from at least six animals). ( c ) Probability histogram of intercoactivity intervals for multiparas exposed to Control and 18-alpha-glycerrhitinic acid (AGA) 20 μM. GJ blockade with AGA results in reversion to a primipara intercoactivity interval distribution due to abolition of cell synchrony ( n =8 slices from three animals). ( d ) Probability histogram of intercoactivity intervals for multiparas suckled by a reduced number of pups during the first lactation. Prior exposure to a reduced suckling stimulus disrupts appearance of coactivity peaks in multiparas as shown by a non-Gaussian distribution of intercoactivity intervals ( n =13 slices from five animals). ( e ) Tissue output in the form of prolactin (PRL) secretion markedly increases as a function of lactational experience (** P <0.01 versus nullipara (NP), # # P <0.01 versus primipara (PP); Kruskal–Wallis test) and this can be reversed by exposing multiparas to reduced demand during the first lactation (NS, nonsignificant versus PP; Kruskal–Wallis test; n =6–19 animals). Values represent mean±s.e.m.± Full size image The results of this study indicate that, by virtue of their network organization, pituitary lactotrophs respond to lactation with increases in coordinated cell–cell communication, FC and tissue output. Following weaning, the lactotroph population is able to maintain FC patterns for weeks to months, a signature of long-term experience-dependent plasticity as commonly encountered in cells comprising the brain [5] . Remarkably, in a manner reminiscent to that observed in neurons [3] , [4] , the lactotroph population retains FC through changes in the extent and strength of cell–cell communication, allowing repeat challenge with identical stimulus to be met with evolved network behaviour and incremental improvements in tissue function. Specifically, long-lasting experience-dependent changes were permitted by the large-scale arrangement of lactotrophs into a highly plastic GJ-linked network, allowing the formation of long-distance functional connections through the entrainment of cell activity. Suggesting that intercellular communication was facilitated by the electrically driven propagation of regenerative Ca 2+ signals were the observations that two-dimensional conduction velocity was rapid (likely to be underestimated given the complex three-dimensional arborization of the lactotroph network), and Ca 2+ -spike amplitude was similar in entrained cells. It is unlikely that substrates such as inositol triphosphate are implicated in lactotroph network signalling events, as we have previously shown that intracellular signalling molecules propagate at under 15 μm s −1 in similar pituitary slice preparations [30] . The presence of quiescent neighbouring cells in the FC maps is presumably a consequence of network information exchanges through three-dimensional chains of GJ-coupled lactotrophs. Indeed, preferential communication paths that reflect differing GJ transfer efficiencies may account for the inability of immediately juxtaposed cells to entrain and coordinate activity when viewed as a two-dimensional optical section [33] . Of note, intercellular communication within the lactotroph network was highly plastic due to effects of suckling on SC and GJ coupling, leading not only to transient increases in coordinated population activity, but also longer-term changes in FC. Given that increases in SC and GJ signalling strength were temporally associated with the appearance of multiple well-connected nodes, it is reasonable to speculate that these tuneable mechanisms may provide a means to encourage and maintain information flow between node and follower cells during and after demand. Although lactation is associated with lowered dopamine neuron tone [25] , [26] , the effects of suckling on intercellular communication and network function seem to require the permissive actions of other hypothalamic and/or peripheral signals, as D2-receptor antagonism was without effect. Other potential candidates include oxytocin- and vasopressin-producing neurons, which are known to be targeted by suckling to impact lactotroph activity [34] , [35] , [36] . Crucially, suckling-evoked changes in lactotroph network connectivity were detectable for upto 3 months following cessation of the original lactation episode. Whereas similar plastic responses have been documented in cells belonging to a range of other tissues outside of the central nervous system (for example, skeletal muscle), they are not persistent insofar as reversion tends to occur if there is significant delay between re-presentation of stimulus [37] , [38] . The observation that lactotroph output displays long-term plasticity in response to suckling stimulus adds a hitherto unknown element to neuroendocrine adaptation of the maternal brain. PRL is a pleiotropic hormone capable of affecting neural circuits involved in the control of centrally mediated functions such as feeding, stress and reproduction, all of which are altered during pregnancy and lactation when hormone concentrations peak [39] , [40] . Functional adaptation of lactotroph network activity may therefore have wide-ranging repercussions for many downstream effectors, modifying physiology and behaviour accordingly when females undergo one or more lactations. Moreover, multiparous dams show improvements in spatial memory that can be reversed following intracerebroventricular injection of an oxytocin receptor antagonist [41] , [42] . It is not unfeasible that the persistent changes in spatial memory are programmed through the effects of PRL on PRL-receptor-expressing oxytocin neurons [43] , [44] , a population which has previously been shown to undergo long-term priming in response to repeated demand [12] . More broadly, these findings raise the possibility that other members of the endocrine system may possess emergent experience-dependent responses at the population level. Pancreatic β-cells are potential candidates as they are organized into ephrin and GJ-linked cell ensembles [45] , [46] , mount highly coordinated responses to stimulus [47] and display marked plasticity throughout lifespan [48] , [49] . Furthermore, gut endocrine cells, which respond to nutritional status by secreting metabolic-signalling peptides such as ghrelin and GLP-1 [50] , [51] , merit revisiting. Although traditionally regarded to be part of the diffuse endocrine system [52] , functional tissue organization may suggest a role for experience-dependent plasticity in determining the long-term hormonal and homeostatic responses to repeated caloric demand/insult. In summary, this study shows that emergent experience-dependent responses are a feature of lactotrophs arranged as a network in the mammalian pituitary gland, allowing functional adaptation of hormone release following repeat stimulation. As such, these results provide important insights into how endocrine organs that mediate important body processes function at the population level. Animals Transgenic mice expressing DsRed under the control of the PRL promoter were used in all experiments [22] , [31] . In studies involving nulliparas (virgin animals), only animals displaying metestrous/diestrous or oestrous were used (vaginal cytology followed for at least two consecutive cycles). For lactating studies, females were mated with wild-type CB57/BL6 males and killed between days 8 and 12 of lactation. For weaning studies, dams were weaned on day 15 of lactation and killed either 3 weeks or 3 months later. For studies involving multiparas (second lactation), animals were re-mated 3 weeks following weaning and experiments performed as for the first lactation. For studies of reduced demand, pups were removed immediately postpartum such that only three pups continued to suckle. A proportion of these dams were weaned and subjected to a second, normal lactation. In all experiments, mice were killed by rapid decapitation before extraction of the pituitary gland and preparation as previously described [8] , [9] . Plasma samples were used for measurement of PRL concentrations. PRL-DsRed/GH-eGFP animals were generated by crossing PRL-DsRed with GH-eGFP mice [53] . All animal studies complied with the animal welfare guidelines of the European Community, and/or UK Home Office guidelines, as appropriate (agreement no. 34.128). Drug treatment regimes are detailed in the Supplementary Methods . Calcium imaging For multicellular calcium (Ca 2+ ) imaging, pituitary slices (150 μm) were incubated (37 °C, 95% O 2 /5% CO 2 ) for 1 h in fura-2-AM (20 μM) diluted with a mixture of dimethylsulphoxide (0.01%, wt/vol) and pluronic acid (0.005%, wt/vol; all Invitrogen) in Ringers solution (125 mM NaCl, 2.5 mM KCl, 1.25 mM NaH 2 PO 4 , 26 mM, NaHCO 3 , 12 mM glucose, 2 mM CaCl 2 and 1 mM MgCl 2 ). Changes in cytosolic Ca 2+ were measured using a multibeam two-photon system (Trimscope). For all experiments, approximately 300×300 μm field (2×2 binning) representing one-quarter of the adenohypophysis was imaged in 64-beam mode using a low magnification, infrared-adjusted water-immersion objective (×20, NA 0.95 Plan Fluorite, Olympus). A femtosecond-pulsed laser (Ti:Sapphire; Coherent) provided wavelengths of 780 nm and 970 nm to excite fura-2 and DsRed, respectively. Images were captured by a 14-bit, 512×512 pixel back-illuminated EM-CCD camera (Andor) and emitted signals recorded from 468 to 552 nm for fura-2 and 573 to 613 nm for DsRed. Lambda scans were performed to ensure that there was no overlap of the emitted fluorescence signals. During this time, slices were incubated at 36 °C and continuously irrigated with Ringers aerated with 95% O 2 /5% CO 2 and supplemented with 1 mM ascorbic acid (Sigma-Aldrich). In ours and other hands [54] , Ca 2+ -indicator uptake is limited to the first two cell layers of the pituitary gland ( Supplementary Fig. S8a and b ). To avoid artefacts due to recording at the cut surface, cells were consistently imaged at 10–15 μm depth (that is, second cell layer). This avoided uncertainties regarding simultaneously capturing Ca 2+ signals from fura-2-loaded cells below the imaged plane. Furthermore, at an excitation wavelength of 780 nm, using a ×20 objective (0.95 NA) and EM-CCD, the axial resolution of the microscope in multibeam mode is 1.42±0.02 μm ( ∼ 10% higher at 15-μm depth) [55] . In agreement with this value, the axial resolution of our system was 1.55±0.07 μm as measured using the point spread function of Tetraspeck beads (Invitrogen) embedded in agarose. Therefore, it is unlikely that fura-2-expressing cells above the second layer were inadvertently recorded. In all cases, we confirmed that a single-DsRed cell was identified using a region of interest by consulting the three-dimensional stacks acquired immediately before each experiment. Finally, upto a threefold difference in fura-2 intensity was detected between lactotrophs. This was likely caused by loading discrepancies as opposed to major differences in baseline Ca 2+ levels. Indeed, in DsRed-expressing cells that displayed decreased intracellular Ca 2+ levels in response to zero (0 mM) Ca 2+ (+EGTA 5 mM; n =3 slices/3 animals), the distribution of fura-2 intensity values remained unaltered versus normal Ca 2 concentrations ( Supplementary Fig. S9a and b ). In the case of similar cell loading, but differing baseline/resting Ca 2+ concentrations, we would have expected a shift in the fura-2 intensity cumulative frequency histogram under zero Ca 2+ conditions ( Supplementary Fig. S9b , red dashed line). Importantly, Ca 2+ -spiking profiles were not affected by fura-2 intensity, demonstrating that the observed differences in fura-2-loading levels were not influencing cell activity (for example, due to Ca 2+ buffering; Supplementary Fig. S9c ). In addition, there were no significant differences in the distribution of fura-2 intensities between virgin and lactating animals ( n =5 slices/5 animals), indicating that fura-2 loading, and any effects of this upon cell activity, was unaltered by physiological state ( Supplementary Fig. S9d ). Prolactin radioimmunoassay Plasma PRL concentrations were measured using specific radioimmunoassay and reagents from The National Institute of Diabetes and Digestive and Kidney Diseases (NIDDK), as previously described [56] . Cell dispersion Cells were dispersed using trypsin, dispase, collagenase and DNAase as described in the Supplementary Methods . Multiphoton and confocal imaging of fixed tissue Tissues were fixed overnight using 4% paraformaldehyde before being subjected to imaging, as outlined in the Supplementary Methods . Electron microscopy Endocrine cells were identified on the basis of their secretory granule populations, organelle structure, nucleus size and chromatin characteristics. Immunogold labelling for PRL, luteinizing hormone and GH was also performed to assist with the identification of lactotrophs, gonadotrophs and somatotrophs, respectively. Ultrathin sections were incubated for 2 h with rabbit anti-rat PRL (1:5,000), guinea-pig anti-rat luteinizing hormone (1:3,000) or monkey anti-rabbit GH (1:5,000; from NIDDK) and were subsequently incubated for 1 h with protein A–15 nm gold complex (British Biocell). The number of intercellular junction-type contacts between lactotrophs and other pituitary cell types was noted (40 lactotrophs/4 animals). Dye transfer assay Dye transfer studies were performed using a conventional light microscope (Zeiss Axioplan) equipped with differential interference contrast. Dye was introduced into lactotrophs using sharp microelectrodes. As some minor bleed of the DsRed signal into the yellow channel ( ∼ 540 nm) was experienced under epifluorescent conditions, the ultraviolet-excitable GJ-permeable compound, Cascade Blue (5% in LiCl 150 mM, pH 7; molecular weight=548.29 Da; neutral; Invitrogen), was used to ensure accurate dye tracing. The extent and nature of cell–cell coupling was estimated directly online by counting the number and type of cell that received dye, as previously described [33] . AGA (20 μM; Sigma-Aldrich) was used as a GJ blocker [57] . To confirm passage of dye to cells outside of the focal plane, a proportion of slices were fixed and subjected to confocal imaging ( Supplementary Fig. S10a ). No differences in the transfer of Cascade Blue or its smaller, anionic counterpart, Alexa-350 (Invitrogen), were observed in lactating animals ( n =21 injected cells/6 slices). This suggests that lactotroph–lactotroph GJ pore size and charge selectivity is not a limiting factor for dye transfer, at least between molecular weights of ∼ 349 and ∼ 548 Da ( Supplementary Fig. S10b and c ). Electrical stimulation of lactotroph activity As lactotrophs display high levels of spontaneous activity under all states investigated, accurate discrimination of simultaneous Ca 2+ rises under resting conditions were precluded following local voltage stimulation. Therefore, dopamine (100 nM in 1 mM ascorbic acid; Sigma-Aldrich), a lactotroph-specific hyperpolarizing agent [58] , was used to reduce network activity. Patch pipettes (4–8 MΩ) containing fluorescein isothiocyanate-Ringer's were lowered onto DsRed-expressing cells using epifluorescence before switching to two-photon excitation. Lactotroph membrane contact was verified in the recording plane using both the fluorescein isothiocyanate emission as well as the dark shadow cast by the pipette tip. Subsequently, fura-2 signals were recorded at 6–7 Hz for a brief control period before injection of voltage (0.5–5 V) for 500 ms, as previously described [30] . Although dopamine decreases Ca 2+ –current amplitude in lactotrophs [58] , electrical stimulation was sufficient to trigger Ca 2+ spikes in stimulated cells. Cells were only included in analyses if the cell in direct contact with the pipette responded to voltage-induced depolarization by firing a Ca 2+ spike. Entrained DsRed-positive cells were identified on the basis of at least a 20% increase in intracellular Ca 2+ levels, which lagged behind that of the stimulated cell. Weaned animals were used in all studies due to their extensive GJ coupling and relatively low levels of spontaneous lactotroph activity. It should be noted that the number of entrained cells was likely underestimated due to the effects of dopamine on membrane excitability. Correlation and connectivity analyses Correlation analyses were performed using signal binarization and randomized matrix analysis as detailed [59] . Frequency and connectivity analyses were performed using the fast Fourier transform and Euler characteristic, respectively. All analyses are described in the Supplementary Methods . Statistical analysis In all cases, data distribution was tested using a D'Agostino omnibus normality test. To account for non-normality and unequal sample sizes, the effects of treatment and physiological state on exponent value ( γ ), correlated cell pair number, cell volume, pituitary volume occupied by lactotrophs, PRL output and connectivity were assessed using either Mann–Whitney U -test or Wilcoxon signed-rank test, or where multiple variables were considered, Kruskal–Wallis test followed by Dunn's post-hoc test. The effects of physiological state on Ca 2+ -spiking frequency and fura-2 intensity distribution were assessed using two-way analysis of variance (followed by Bonferroni's post-hoc test; data normally distributed). In all cases, at least three independent experiments were tested and changes were considered significant at P <0.01 and P <0.05. Values are presented as either mean±s.e.m. or median±interquartile range. Unless otherwise stated, MATLAB (Mathworks), Igor (WaveMetrics) and Graphpad Prism (Graphpad Software) were used for all analyses. How to cite this article: Hodson, D.J. et al . Existence of long-lasting experience-dependent plasticity in endocrine cell networks. Nat. Commun. 3:605 doi: 10.1038/ncomms1612 (2012).